Ultrafast magnetization enhancement in metallic multilayers driven by superdiffusive spin current Uncovering the physical mechanisms that govern ultrafast charge and spin dynamics is crucial for understanding correlated matter as well as the fundamental limits of ultrafast spin-based electronics. Spin dynamics in magnetic materials can be driven by ultrashort light pulses, resulting in a transient drop in magnetization within a few hundred femtoseconds. However, a full understanding of femtosecond spin dynamics remains elusive. Here we spatially separate the spin dynamics using Ni/Ru/Fe magnetic trilayers, where the Ni and Fe layers can be ferro- or antiferromagnetically coupled. By exciting the layers with a laser pulse and probing the magnetization response simultaneously but separately in Ni and Fe, we surprisingly find that optically induced demagnetization of the Ni layer transiently enhances the magnetization of the Fe layer when the two layer magnetizations are initially aligned parallel. Our observations are explained by a laser-generated superdiffusive spin current between the layers. One of the major roadblocks for continued progress in nanoelectronics is energy dissipation caused by the flow of electrical current. Encoding data in electron spin, rather than charge, promises a new route for technology with the potential to dramatically reduce these energy requirements. A current grand challenge in this area is to control the static and dynamic behaviour of spins and spin ensembles. Spin dynamics is in-itself of fundamental interest for understanding spin–photon–charge–phonon interactions and their complex interplay on femtosecond to picosecond timescales. The potential to rapidly manipulate spins was first demonstrated in a pioneering experiment [1] on Ni that observed that the magnetization of 3 d ferromagnets can be optically quenched within 50–300 fs after excitation by a femtosecond laser pulse [2] , [3] . This ultrafast demagnetization is then followed by a slower magnetization recovery on picosecond timescales. Optically induced magnetization reversal has also been demonstrated using circularly polarized light [4] . A number of distinct models have been proposed to describe how laser excitation can couple so quickly to the spins, given that the light itself does not directly exert a significant torque on the electron spins. Most of these models are based on phonon-, electron- and magnon-mediated spin–flip processes [5] , [6] , [7] , [8] , [9] , direct laser-induced spin–flips [10] or relativistic spin–light interaction [11] . Most recently, a new model based on superdiffusive spin transport has been proposed [12] , [13] . The variety of these distinct interpretations suggests that several physical mechanisms may govern femtosecond spin dynamics even in a simple elemental magnet. The physics becomes even more intriguing for heterogeneous magnetic systems, such as magnetic compounds [14] , alloys [15] , [16] and exchange-coupled layered structures. Several sophisticated experiments have recently employed ultrashort soft X-ray pulses from synchrotron [2] , [15] or laser-driven high-harmonic (HHG) light sources [3] , [16] , [17] to disentangle the various processes using element-specific demagnetization techniques. This has been achieved by monitoring the absorption or reflection of light tuned to inner-shell absorption edges of magnetic materials. Using these new capabilities, unexpected new spin dynamics can be uncovered—for example, even in a strongly coupled ferromagnetic permalloy (Fe 20 Ni 80 ), the magnetization of Fe quenches faster than the Ni magnetization for a time shorter than the characteristic energy/time equivalent of the exchange coupling energy of the alloy [16] . In magnetic multilayers, magnetization dynamics has been previously studied on nanosecond to picosecond timescales [18] , [19] , [20] . However, accurately explaining how multilayer systems demagnetize on femtosecond timescales has proven challenging. Recent exciting experiments optically pumped layered magnetic structures using femtosecond lasers [21] , [22] and inferred the resulting spin transport dynamics using visible probe light. Here we exploit the combination of simple magnetic multilayer structures and the powerful capability of our HHG probe to simultaneously monitor layer-specific magnetization dynamics. We study a Ni/Ru/Fe trilayer stack under conditions where superdiffusive spin transport is the dominant process determining spin dynamics on the fastest timescales. By optically exciting the stack with femtosecond laser pulses and probing the resulting magnetization dynamics in the Ni and Fe layers simultaneously but element-selectively at the 3 p (M) absorption edges of Ni (66 eV) and Fe (52 eV), we directly observe magnetization dynamics in individual layers. Remarkably, we find that the femtosecond spin dynamics of the individual Ni and Fe layers depends on the relative alignment of their initial magnetization directions: ultrafast excitation and demagnetization of the Ni layer transiently enhances the magnetization of the buried Fe layer when their magnetizations are initially aligned parallel to each other, whereas the magnetization of the Fe layer decreases if its initial magnetization is antiparallel to that of Ni. These findings can be explained consistently by large laser-generated superdiffusive spin currents [12] , [13] . In this physical picture, superdiffusion of excited spin majority electrons from the Ni layer, through the Ru layer and into the buried Fe layer can transiently increase or decrease the magnetization in Fe depending on its relative spin alignment with respect to Ni (which can be controlled by the external magnetic field and the thickness of the Ru spacer layer). Multilayer fabrication and characterization Our samples consist of Al(3 nm)/Ni(5 nm)/Ru( x )/Fe(4 nm)/Ta(3 nm) layers (see Methods ), where the Ni/Ru/Fe trilayer forms an interlayer exchange-coupled magnetic system ( Fig. 1 ). The top Si 3 N 4 grating structure serves as a grating spectrometer to spectrally disperse the extreme ultraviolet (XUV) HHG radiation spanning from approximately 20 to 72 eV. The magnetism in our samples was carefully characterized using a superconducting quantum interference device (SQUID) magnetometer. These data (see Fig. 2 ) show the influence of the Ru spacer thickness on the interlayer exchange-coupling between Ni and Fe layers: a 1 nm thick Ru layer results in a ground-state ferromagnetic coupling for Ni and Fe, which changes to antiferromagnetic coupling for a 1.5 nm Ru layer thickness. 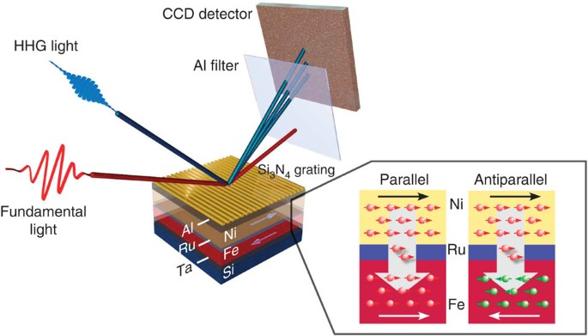Figure 1: Experimental setup and the multilayer sample schematics. The magnetization of the Al/Ni/Ru/Fe multilayer samples is probed by XUV high harmonics at the 3pabsorption edges of Fe and Ni. The Si3N4grating on top of the layers spectrally separates the XUV high harmonic beams that are then detected by an X-ray CCD detector. The pump laser light absorbed in the thin Al and Ni layers results in a spin current (marked by grey arrow in the inset) that travels through the non-magnetic Ru spacer layer into the Fe layer. The magnetization of the Fe layer increases or decreases depending on its orientation relative to Ni. The inset illustrates schematically the relative magnetization of the Ni and Fe layers (thin black and white arrows), the majority spin alignment in the layers (red and green circles) and the flow of the spin current (large grey arrow). Figure 1: Experimental setup and the multilayer sample schematics. The magnetization of the Al/Ni/Ru/Fe multilayer samples is probed by XUV high harmonics at the 3 p absorption edges of Fe and Ni. The Si 3 N 4 grating on top of the layers spectrally separates the XUV high harmonic beams that are then detected by an X-ray CCD detector. The pump laser light absorbed in the thin Al and Ni layers results in a spin current (marked by grey arrow in the inset) that travels through the non-magnetic Ru spacer layer into the Fe layer. The magnetization of the Fe layer increases or decreases depending on its orientation relative to Ni. The inset illustrates schematically the relative magnetization of the Ni and Fe layers (thin black and white arrows), the majority spin alignment in the layers (red and green circles) and the flow of the spin current (large grey arrow). 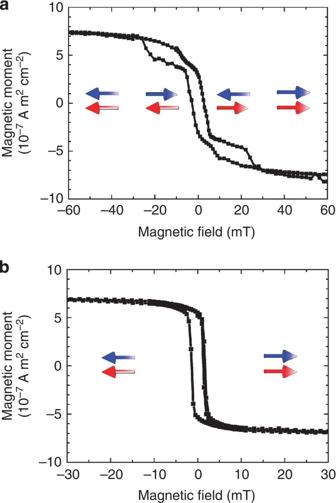Figure 2: Magnetic hysteresis loops. The magnetic moment of the Ni(5 nm)/Ru(x)/Fe(4 nm) trilayers, wherex=1 nm and 1.5 nm, was measured by a SQUID magnetometer at 290 K. The Fe and Ni layers in the trilayer with a Ru thickness of 1.5 nm (a) are antiferromagnetically coupled in zero external magnetic field, whereas they are ferromagnetically coupled in the 1 nm thick Ru trilayer (b). The red and blue arrows show the magnetizations of Fe (red) and Ni (blue) layers indicating the relative magnetization orientation within a specific magnetic field range. Full size image Figure 2: Magnetic hysteresis loops. The magnetic moment of the Ni(5 nm)/Ru( x )/Fe(4 nm) trilayers, where x =1 nm and 1.5 nm, was measured by a SQUID magnetometer at 290 K. The Fe and Ni layers in the trilayer with a Ru thickness of 1.5 nm ( a ) are antiferromagnetically coupled in zero external magnetic field, whereas they are ferromagnetically coupled in the 1 nm thick Ru trilayer ( b ). The red and blue arrows show the magnetizations of Fe (red) and Ni (blue) layers indicating the relative magnetization orientation within a specific magnetic field range. Full size image Static magnetic asymmetry The magneto-optical response of our trilayers is measured via the transverse magneto–optical Kerr effect (T-MOKE) in XUV spectral range [23] , [24] , [25] (see Supplementary Methods for a more detailed description). Magnetic asymmetry can be defined as where I r ( H ↑ ) and I r ( H ↓ ) denote the intensities of the reflected light as the externally applied magnetic field H is reversed in direction. Measuring I r ( H ) for these two opposite field directions gives an artifact-free and sensitive measurement of the magnetic state [16] , [17] , [26] . The resonantly enhanced static magnetic asymmetry at the Fe and Ni 3p absorption edges (52 and 66 eV, respectively) can be clearly assigned to the magnetic state of the Fe and Ni layers, as shown in Fig. 3 . For our Ni/Ru/Fe trilayer, the amplitude of the magnetic asymmetry is around 10% at the Fe absorption edge and 20% at the Ni 3 p edge. By adjusting the external magnetic field from 0 to ±60 mT, we can tune the trilayers into two well-defined magnetic states: one with parallel orientation of the Ni and Fe magnetizations and one with antiparallel orientation. A comparison of the magnetic asymmetries corresponding to the two states shows that the relative sign of the Ni and Fe asymmetries reverses in these two cases. 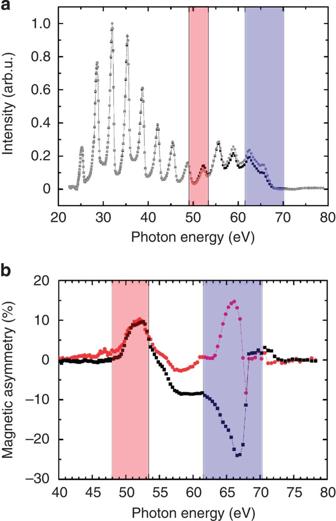Figure 3: High harmonics and magnetic asymmetry spectra. (a) Spectra of high harmonics reflected from the sample depend on the orientation of the external magnetic field (H↑or H↓). The spectra are taken for parallel alignment of the Ni and Fe magnetizations for H↑(black squares) and H↓(grey circles). The spectra differ at the 3pabsorption edges of Ni (blue-coloured area) and Fe (red-coloured area). (b) Fe and Ni magnetic contributions can be separated in the magnetic asymmetry calculated from high harmonics spectra (equation (1)). The 3pabsorption edges of Fe and Ni are marked by red- and blue-coloured areas. For parallel alignment of the Ni and Fe magnetizations the Ni and Fe asymmetry peaks have different signs (black squares) whereas for the antiparallel alignment (red circles) the sign of the Ni asymmetry peak reverses. Figure 3: High harmonics and magnetic asymmetry spectra. ( a ) Spectra of high harmonics reflected from the sample depend on the orientation of the external magnetic field (H ↑ or H ↓ ). The spectra are taken for parallel alignment of the Ni and Fe magnetizations for H ↑ (black squares) and H ↓ (grey circles). The spectra differ at the 3 p absorption edges of Ni (blue-coloured area) and Fe (red-coloured area). ( b ) Fe and Ni magnetic contributions can be separated in the magnetic asymmetry calculated from high harmonics spectra (equation (1)). The 3 p absorption edges of Fe and Ni are marked by red- and blue-coloured areas. For parallel alignment of the Ni and Fe magnetizations the Ni and Fe asymmetry peaks have different signs (black squares) whereas for the antiparallel alignment (red circles) the sign of the Ni asymmetry peak reverses. Full size image Magnetization dynamics To capture spin transport and magnetization dynamics in our trilayer, the samples are excited with femtosecond pump laser pulses of 1.6 eV photon energy. The magnetization in the individual layers was then captured simultaneously by monitoring the amplitude of the T-MOKE magnetic asymmetry as a function of time delay. To estimate the amount of the pump light reaching the individual layers, we performed a self-consistent 2×2 matrix calculation of the optical properties for the full metallic layer stack for our experimental conditions. We find that the combination of the Al cap and Ni layer together absorbs >58% of the incident light—about 2.5 times as much as the Fe layer. Generally, as in all optical pump-probe experiments, it is possible that the magneto–optical signal is affected by the hot electrons, in which case the signal would also change sign with switching the magnetization. However, the fact that changing the relative magnetization direction of the Fe layer relative to the Ni layer (see below) causes an increase or decrease of the observed Fe magnetization, rules out such measurement artifacts. In addition, in a previous publication [17] we showed that the nonmagnetic contribution to the asymmetry parameter is small (0.2%) compared with the amplitude of demagnetization (20%), demonstrating that XUV T-MOKE can sensitively probe element-selective spin dynamics. The layer-selective time traces of the magnetic asymmetries at the 3 p absorption edges of Fe and Ni, at fluencies of F ≈2 mJ cm −2 , are plotted in Fig. 4a,b . Similar to earlier experiments [1] , [2] , [3] , [5] , we observe a magnetization quenching in the Ni layer of the stack. Surprisingly, however, we also observe either an enhancement or reduction of the Fe magnetization depending on the relative magnetization orientation of the Ni and Fe layers (see Fig. 4a,b ): if the Fe and Ni layers are initially oriented antiparallel, then the magnetization of both Ni and Fe decreases. On the other hand, if the two layers are oriented parallel by an external magnetic field, we observe that the Fe magnetization increases 15% above its equilibrium value on a similar timescale. In a second layer stack with Ni(5 nm)/Ru(1 nm)/Fe(4 nm), where the Ni magnetization only aligns parallel to the Fe one ( Fig. 4c ), we observe again an enhancement in the Fe magnetization after laser excitation. 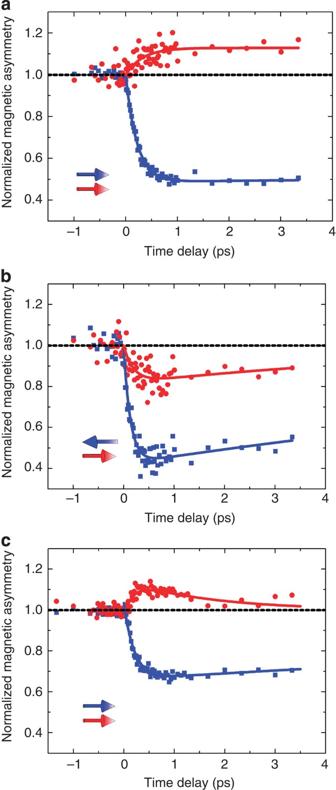Figure 4: Experimentally measured time- and layer-resolved magnetization. The time-resolved magnetization of the Fe and Ni layers in the Ni(5 nm)/Ru(1.5 nm)/Fe(4 nm) trilayer for the parallel (a) and antiparallel (b) magnetization alignment and in the Ni(5 nm)/Ru(1 nm)/Fe(4 nm) trilayer (c) for the parallel magnetization alignment. The data have been extracted by integrating the magnetic asymmetry signal over the 3pabsorption edges of Fe and Ni, as indicated by the red- and blue-coloured areas inFig. 3, respectively, and normalizing to the magnetic asymmetry values before the time zero (black broken line). The magnetic asymmetry at the Fe 3pabsorption edge anomalously increases for the parallel (a,c) and decreases for antiparallel magnetic orientation of Ni and Fe layers (b). For the Ni(5 nm)/Ru(1 nm)/Fe(4 nm) trilayer, only parallel magnetization orientation is possible due to ferromagnetic coupling. The curves are least square fits toSupplementary Equation (S2). Figure 4: Experimentally measured time- and layer-resolved magnetization. The time-resolved magnetization of the Fe and Ni layers in the Ni(5 nm)/Ru(1.5 nm)/Fe(4 nm) trilayer for the parallel ( a ) and antiparallel ( b ) magnetization alignment and in the Ni(5 nm)/Ru(1 nm)/Fe(4 nm) trilayer ( c ) for the parallel magnetization alignment. The data have been extracted by integrating the magnetic asymmetry signal over the 3 p absorption edges of Fe and Ni, as indicated by the red- and blue-coloured areas in Fig. 3 , respectively, and normalizing to the magnetic asymmetry values before the time zero (black broken line). The magnetic asymmetry at the Fe 3 p absorption edge anomalously increases for the parallel ( a , c ) and decreases for antiparallel magnetic orientation of Ni and Fe layers ( b ). For the Ni(5 nm)/Ru(1 nm)/Fe(4 nm) trilayer, only parallel magnetization orientation is possible due to ferromagnetic coupling. The curves are least square fits to Supplementary Equation (S2) . Full size image Superdiffusive spin transport This first observation of an ultrafast magnetization enhancement in the Fe layer can be explained by superdiffusive spin transport [12] , [13] (see also Supplementary Discussion ), taking place on timescales comparable to the demagnetization processes explored in earlier works [1] , [2] , [3] , [5] . The mechanism we propose for enhancement of the magnetization is based on filling of majority spin states above the Fermi energy in the Fe layer by majority spins coming from Ni. This leads to a transient magnetization increase in the Fe layer, above its maximum value defined by the Curie curve at T =0 K. The increase in the magnetic signal from the Fe layer is a result of a strong asymmetry in the spin-dependent hot-electron lifetimes in magnetic materials and, hence, the transport properties of the hot majority and minority spin carriers [27] , [28] , [29] within the Ni and Fe layers. Excited minority spin electrons originating in the optical excitation in both the Al and Ni layers have much shorter lifetimes when passing via superdiffusion through the Ni layer, and are therefore stopped before they can reach the Fe layer. Conversely, majority-spin electrons have much longer lifetimes in Ni and are able to reach the Fe layer by superdiffusion. Solving the superdiffusion spin-transport equation (see Methods ) for electrons excited by a laser pulse of 25 fs and 1.6 eV photon energy in the Al, Ni and Fe layers, we predict the transient, layer-specific, normalized magnetizations shown in Fig. 5 . The transient response of the Fe layer depends strikingly on the initial relative alignment of the Ni and Fe layers: for antiparallel magnetization alignment, the stream of spin-majority electrons decreases the net magnetization in the Fe layer by increasing the amount of spin-minority electrons in Fe. Conversely, for parallel configuration, the superdiffusive spin current of spin majority electrons through the interface increases the number of spin-majority electrons in Fe, thus increasing the net Fe magnetization and causing opposite polarities in the femtosecond magnetization response of Ni and Fe layers. 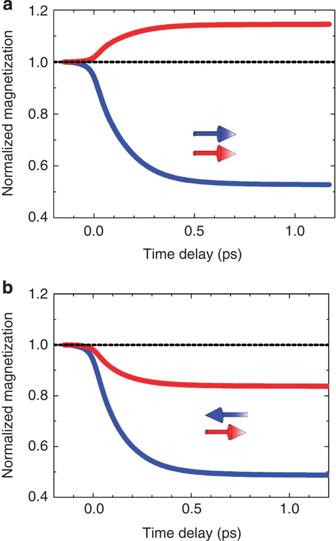Figure 5: Calculated time- and layer-resolved magnetization. In our model, laser-induced ultrafast demagnetization of the Ni layer (blue curves in (a) and (b)) generates superdiffusive spin currents that increase the Fe magnetization for parallel orientation (a) (red curve), whereas decreasing the Fe magnetization for antiparallel alignment (b) (red curve). The strengths and timescales of demagnetization and magnetization agree well with the measured data. Figure 5: Calculated time- and layer-resolved magnetization. In our model, laser-induced ultrafast demagnetization of the Ni layer (blue curves in ( a ) and ( b )) generates superdiffusive spin currents that increase the Fe magnetization for parallel orientation ( a ) (red curve), whereas decreasing the Fe magnetization for antiparallel alignment ( b ) (red curve). The strengths and timescales of demagnetization and magnetization agree well with the measured data. Full size image Several competing processes have been proposed for magnetization dynamics on ultrafast timescales [5] , [6] , [7] , [8] , [9] , [10] , [11] , [12] , [13] . For the trilayer systems explored here, we find that the observed magnetization dynamics in the Ni and buried Fe layer is consistent with superdiffusion of excited spin-majority electrons that originate in the Al and Ni layers. The experimental data ( Fig. 4a,b ) agree well with theoretical predictions of superdiffusive spin transport ( Fig. 5a,b )–both in terms of the timescales as well as the magnitudes of the demagnetization (~15% for Fe and ~50% for Ni) and anomalous magnetization increase in Fe (~15%). We note that we have not included spin dissipation channels such as electron–phonon [5] and electron–electron [7] spin–flip scattering in our model. This excellent agreement between theory and experiment thus shows that superdiffusion is the dominant process for the observed spin dynamics in the Ni and Fe layers under the chosen experimental conditions. The anomalous enhancement of the Fe magnetization is most prominent at relatively low excitation fluence, below F ≈2.0 mJ cm −2 . We find that at higher fluence, direct optical excitation of the Fe layer becomes the dominant source of demagnetization, that is, by increasing the excitation fluence to F ≈2.7 mJ cm −2 , we observe the Fe magnetization to decrease after excitation, even when the Ni and Fe magnetizations are parallel (see Supplementary Fig. S2 ). This observation confirms theoretical predictions that the superdiffusive spin current saturates at high excitation powers [12] , [13] . Conversely, when we reduce the pump fluence to F ≈1.3 mJ cm −2 , we again observe an increase or decrease of magnetization in Fe due to superdiffusive spin transfer, though the effect is weaker than the response shown in Fig. 4 . In summary, by probing ultrafast spin dynamics in interlayer exchange-coupled magnetic structures with elemental specificity using broad bandwidth coherent high harmonic radiation, we are able to elucidate the contribution of spin superdiffusion to the process of ultrafast spin dynamics. Spin superdiffusion leads to a remarkable and counterintuitive magnetization enhancement in Fe in response to optical pumping when the Ni and Fe magnetizations are initially parallel. Our discovery provides fundamental insight into spin dynamics on femtosecond timescales, and is relevant for identifying the mechanisms underlying ultrafast spin dynamics. We note that our data demonstrate an ultrafast transfer of angular momentum of longitudinal spin through a spin current on subpicosecond timescales. In contrast, previous works demonstrated spin-transfer torque, that is, a transfer of transverse angular momentum between noncollinear spins and a magnetic moment at microwave frequencies [30] , [31] , [32] , [33] , leading to important innovations such as spin–torque magnetic random access memory (RAM) for data storage, spin–torque oscillators for frequency-agile telecommunications, and spin–wave interconnects for spin-based logic. Similarly, we anticipate that superdiffusive spin transfer, which has a considerably larger magnetic moment, can find applications in moving domain walls, switching magnetic nano-elements on subpicosecond timescales or in spin-based electronics operating in the Terahertz frequency range. Sample fabrication and experiment The Al(3 nm)/Ni(5 nm)/Ru( x )/Fe(4 nm)/Ta(3 nm) multilayers (Al on top) with two different Ru thicknesses x =1 nm and 1.5 nm were fabricated on Si substrates by use of ion beam sputtering. To ensure proper crystal texture, samples were grown on top of a thin Ta layer. Al capping layer prevents oxidation of the magnetic layers. The Al is self-passivating, and we expect that the top layer actually consists of approximately 1.5 nm of AlO x that covers 2 nm of metallic Al. The entire structure is sufficiently thin for the XUV light to penetrate through and probe the magnetization of the Fe layer. To generate laser high-order harmonics in the XUV, we used a laser amplifier generating laser pulses with 25 fs duration, 1.9 mJ energy and 1.6 eV photon energy, at 3 kHz repetition rate. Ninety percent of the laser power was focused into a Ne-filled capillary with 150 μm diameter to generate HHG spanning 20–72 eV (ref. 34 ), whereas 10% of the laser energy is used to excite the sample with femtosecond laser pulses with fluencies of, approximately, 2 mJ cm −2 . The estimated duration of the XUV pulses is <10 fs (ref. 16 ), and the XUV light was focused onto the sample using a grazing incidence toroidal mirror. The sample was aligned in the T-MOKE geometry with the magnetization vector of the sample perpendicular to the plane of incidence (see Supplementary Methods ). The p -polarized XUV probe light is reflected at an angle of 45° with respect to the sample surface. The XUV photon energy calibration was performed using the Al filter that serves to shield the CCD (charge-coupled device) detector from direct laser light, and has a well-defined absorption edge at 72.6 eV. Theoretical model and calculations The calculations are based on the superdiffusive spin transport equation [12] , [13] , where n (σ, E , z , t ) is the spin- and energy-dependent density of laser-excited electrons, τ ( σ , E , z ) is the lifetime, and Î are the electron flux and identity operators, Ŝ is an integral operator that computes the source term for next-generation electrons, which result from elastic, inelastic, as well as cascade processes, and S ext (σ, E , z , t ) is the source term containing explicitly the 25 fs pump pulse. The z coordinate is defined as being normal to the layers. The spin- and excitation energy-dependent electronic lifetimes and velocities [27] , [29] , as well as the ratio of excited majority to minority spin electrons [35] , are taken from ab initio calculations. The femtosecond spin dynamics follows from m ( E , z , t )=2μ B [ n (↑, E , z , t )− n (↓, E , z , t )], with m ( E , z , t ) the transient spin moment of excited electrons along the depth profile. The material-dependent M ( t ) is computed as the energy-integrated average of m ( E , z , t ) over an individual layer. Partial reflection at the interfaces between two layers has been included. The energy- and spin-dependent reflectivity has been computed assuming the electrons cross the interface as classical particles, with velocity defined by the band structure in each material. The reflected fraction has been obtained by requiring the conservation of linear momentum upon crossing of the interface. All possible multiple reflection paths are taken rigorously into account. In the calculations of Fig. 5 , we assumed a 5 nm Ni and 4 nm Fe layer with a 3 nm Al capping layer; however, the Ru layer was not included. The Ru layer, being thin and embedded between the two ferromagnetic layers, will have a spin lifetime and velocity different from those of bulk Ru, therefore, the parameters of this thin Ru layer are not well known. However, as the Ru layer is very thin, it has only a marginal role in the transport and can to a good approximation be neglected. How to cite this article: Rudolf, D. et al . Ultrafast magnetization enhancement in metallic multilayers driven by superdiffusive spin current. Nat. Commun. 3:1037 doi: 10.1038/ncomms2029 (2012).